Highly aligned carbon nanotube forests coated by superconducting NbC The formation of carbon nanotube and superconductor composites makes it possible to produce new and/or improved functionalities that the individual material does not possess. Here we show that coating carbon nanotube forests with superconducting niobium carbide (NbC) does not destroy the microstructure of the nanotubes. NbC also shows much improved superconducting properties such as a higher irreversibility and upper critical field. An upper critical field value of ~5 T at 4.2 K is much greater than the 1.7 T reported in the literature for pure bulk NbC. Furthermore, the aligned carbon nanotubes induce anisotropy in the upper critical field, with a higher upper critical field occurring when the magnetic field is parallel to the carbon nanotube growth direction. These results suggest that highly oriented carbon nanotubes embedded in superconducting NbC matrix can function as defects and effectively enhance the superconducting properties of the NbC. In contrast to the power application required of high-temperature superconducting materials [1] , the materials under consideration for hot-electron bolometric superconducting mixers [2] and superconductive radio-frequency cavities [3] require a higher superconducting transition temperature and a high conductivity (or low resistivity) in the normal state, at low temperature. On the basis of this criterion, niobium carbide (NbC), which exhibits high melting point (3,610 °C), good chemical stability, excellent hardness, and superior wear resistance, has been considered as one of the potential materials. Unfortunately, the growth of ceramic-like (or bulk) NbC with desired functionalities has been a big challenge because a reaction temperature above 1,000 °C is generally required. Such a high processing temperature leaves no playground to manipulate the microstructure and/or defect landscape in NbC. In other words, innovative approaches are needed to synthesize NbC with controlled microstructures/defects so that enhanced superconducting properties (such as the irreversibility field, H irr , the highest useful field above which there is no flux pinning and where critical current density is zero), reduced electrical resistivities in the normal state at low temperatures, and improved mechanical strengths can be accomplished for the applications of bolometric mixers and/or coated cavities. Carbon nanotubes (CNTs) are known to be the strongest and stiffest materials in terms of tensile strength and elastic modulus, respectively [4] . Furthermore, the metallic tubes are highly conductive. A successful combination of NbC and CNTs can therefore potentially lead to much improved functionalities and/or create emergent behaviours through coupled competing order parameters. The challenge is, however, to maintain the integrity of individual components after the post processes, because superconducting NbC materials are typically grown at high temperature and CNTs are synthesized in the reduced environment. Here for the first time in the field, we report the integration of superconducting NbC with the highly aligned CNT forests using a chemical solution approach [5] . The formation of superconducting NbC coating on the CNT forests does not destroy the microstructure of CNTs. Importantly, NbC shows much improved superconducting properties such as higher irreversibility field ( H irr ) and upper critical field ( H c2 ). A value of H c2 around 5 T at 4.2 K is much greater than 1.7 T for the pure bulk NbC reported in the literature [6] . Moreover, the aligned CNTs induce anisotropy in H c2 , with higher H c2 , when the magnetic field is parallel to the CNT growth direction. These results suggest that highly oriented CNTs embedded in superconducting NbC can function as defects and effectively enhance the superconducting properties of the NbC. It should be noted that introduction of artificial defects into high-temperature superconducting YBa 2 Cu 3 O 7−x (YBCO) has been broadly investigated to modify the superconducting properties. For example, much improved superconducting properties have been accomplished through introducing columnar defects by high-energy irradiation [7] , [8] and volume defects by inclusion of nanoparticles [9] or of self-assembled, vertically aligned 'bamboo' arrays [9] , [10] . 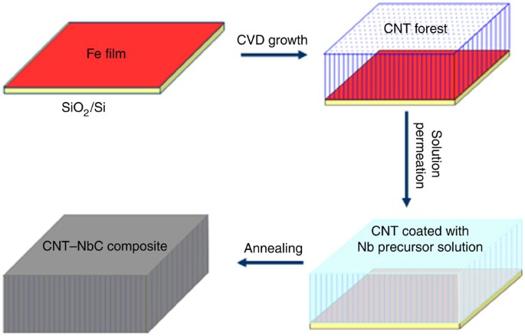Figure 1: The schematic processing steps for the synthesis of CNT–NbC composites. The NbC is the matrix and CNT forest is the second phase material distributed in the matrix. CVD, chemical vapour deposition. Structural properties of CNT–NbC composites Figure 1 shows the schematic drawing of the processing steps to form the CNT–NbC composites. The highly aligned CNT forests were grown on the silicon substrate by a chemical vapour deposition [11] . The CNT forests were then soaked by a homogeneous Nb precursor solution. After detaching the CNT forests from the silicon substrate (simply by peeling off the CNT forest from the Si substrate using a tweezer), we converted the Nb precursor to NbC by annealing the sample under an ethylene environment. Ethylene is also used as the carbon source for the growth of CNT forests [11] . Figure 1: The schematic processing steps for the synthesis of CNT–NbC composites. The NbC is the matrix and CNT forest is the second phase material distributed in the matrix. CVD, chemical vapour deposition. Full size image The integrity of both CNT forests and NbC is maintained after the formation of CNT–NbC composite. 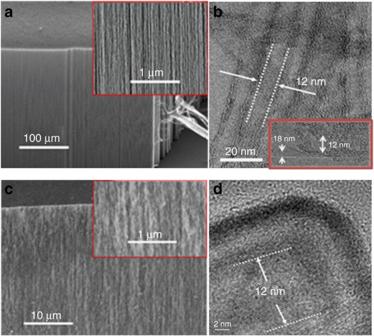Figure 2: Morphology and microstructure of the prepared CNT forest and CNT–NbC composite. (a) SEM image of a highly aligned CNT forest, (b) HRTEM image of CNTs, (c) SEM image of as-synthesized CNT–NbC composite, and (d) HRTEM image of NbC-coated CNT. Insets show the magnified SEM image of CNT forest (a), the high-resolution electron microscopy image of the as-grown multi-wall CNTs (b), and the magnified SEM image CNT–NbC composite (c), respectively. Figure 2 shows the morphologies and the microstructures of the pure CNT and the NbC-coated CNT forests. As can be seen from the scanning electron microscopy (SEM) image shown in Figure 2a , the CNTs prepared by chemical vapour deposition are highly aligned along the growth direction. The enlarged view (inset in Fig. 2a ) clearly shows that the CNTs in the forest are closely packed and homogeneously distributed. The high-resolution transmission electron microscope (HRTEM) image shown in Figure 2b illustrates that the CNTs have multiple walls and an inner diameter of ~12 nm. Detailed HRTEM analysis reveals that the CNT wall thickness is around 1.8 nm (see inset in Fig. 2b ). As compared with the as-grown CNT forest, the whole assembly of NbC-coated CNT forest is even denser as revealed by the SEM image shown in Figure 2c . Furthermore, the cross-section of the NbC-coated CNT forest is quite uniform. The magnified image (inset in Fig. 2c ) clearly shows that well-aligned CNTs are still maintained in the CNT–NbC composite. Figure 2d shows a HRTEM image of NbC-coated CNT. The lattice pattern on the wall matches well with that of the NbC. In addition, a tubular shadow is clearly seen from this HRTEM image. The inner diameter of the tube shadow is around 12 nm that is the same as the diameter of the as-synthesized CNTs shown in Figure 2b . Figure 2: Morphology and microstructure of the prepared CNT forest and CNT–NbC composite. ( a ) SEM image of a highly aligned CNT forest, ( b ) HRTEM image of CNTs, ( c ) SEM image of as-synthesized CNT–NbC composite, and ( d ) HRTEM image of NbC-coated CNT. Insets show the magnified SEM image of CNT forest ( a ), the high-resolution electron microscopy image of the as-grown multi-wall CNTs ( b ), and the magnified SEM image CNT–NbC composite ( c ), respectively. Full size image The full retention of the highly aligned nature of CNT forests in the CNT–NbC composite is confirmed by the X-ray diffraction measurement. To illustrate this, we annealed the Nb precursor-coated CNT forest in pure Ar (in the absence of ethylene) under the same temperature used for the synthesis of CNT–NbC composites. X-ray diffraction θ −2 θ scans (not shown here) revealed (110) Nb and (100) CNT peaks only. The appearance of Nb and CNT peaks only implies that the integrity of the carbon nanotube is retained. In other words, the chemical reaction between Nb and CNT should, if there is any at all, be negligible under such processing conditions. 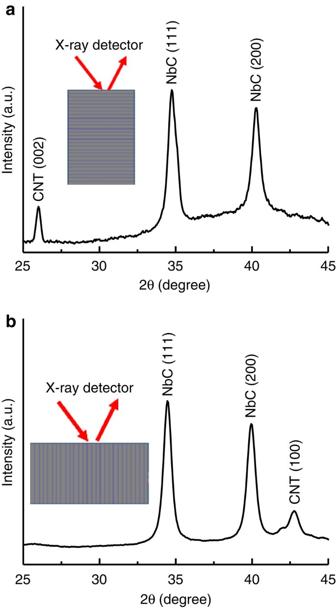Figure 3: X-ray diffraction patterns of as-synthesized CNT–NbC composites. (a) X-ray was irradiated along the side of the sample, and (b) X-ray was irradiated from the top of the sample. Figure 3a shows the typical diffraction pattern of the CNT–NbC composite when the incident X-ray was irradiated along the side of the sample (see the schematic drawing in Fig. 3a ). In addition to diffraction peaks of (111) and (200) from NbC, the (002) peak from the CNTs is visible. On the other hand, when the incident X-ray was irradiated from the top of the sample (see the schematic drawing in the Fig. 3b ), the (100) peak at 42.4° from the CNTs, and the same diffraction peaks from the NbC, are observed as shown in Figure 3b . These results clearly illustrate that the highly aligned CNT forest retains its vertical alignment after the formation of CNT–NbC composite. It should be noted that the interplanar spacing calculated based on the diffraction peaks is a =0.4469 nm for NbC and 0.34 nm for (002) CNT, matching well with the bulk values of NbC and CNT, respectively. Figure 3: X-ray diffraction patterns of as-synthesized CNT–NbC composites. ( a ) X-ray was irradiated along the side of the sample, and ( b ) X-ray was irradiated from the top of the sample. Full size image Superconducting properties of CNT–NbC composites The formation of NbC coating on the CNT forests not only maintains the microstructure of CNTs as discussed above, but more importantly, the CNT–NbC composite shows much improved superconducting properties compared with the pure bulk NbC. First, the CNT–NbC composite shows enhanced H irr and H c2 . 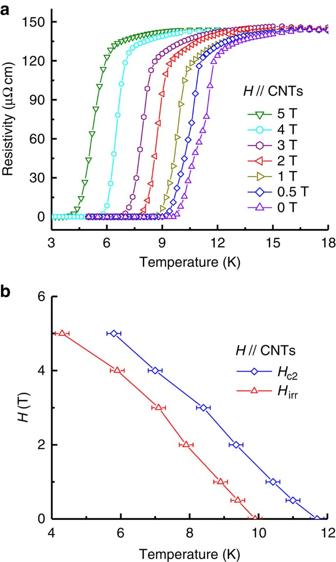Figure 4: Superconducting properties of CNT–NbC composite. (a) Resistivity versus temperature characteristics at different applied magnetic fields, where the magnetic field is parallel to the CNT growth direction, (b) irreversibility field and upper critical field as a function of temperature obtained from those curves, where the irreversibility fieldHirris defined as the field at which theρ/ρN=3% and the upper critical field as the field at which theρ/ρN=80%. Figure 4a shows the resistivity ρ ( T ) versus temperature characteristics as a function of magnetic field ( H ), where the H is applied parallel to the CNT growth direction. Figure 4b shows H irr and H c2 as a function of temperature obtained from those curves. We have used the field at ρ / ρ N =3% to define the H irr , and below H irr , a finite critical current flows, resulting from flux pinning [12] . We have used the ρ / ρ N =80% criterion to define H c2 to avoid the influence of the long tail extending to higher temperatures observed for higher ρ / ρ N fractions, where ρ N is the normal state resistivity near the transition. The H irr value for our CNT–NbC composite reaches as high as 5 T at 4.2 K. The H c2 is even higher. On the basis of our knowledge, these are the highest reported H irr and H c2 for the bulk NbC. Hence, the inclusion of highly aligned CNTs in the NbC significantly improves the performance of the NbC under magnetic field. It should be noted that thin film NbC can show very different superconducting properties, in comparison with its counterpart of bulk NbC. For example, our very thin epitaxial NbC films, grown by polymer-assisted deposition (not shown here), have a similar H irr value as the bulk CNT–NbC composites. Similar to the high-temperature superconductor, YBCO, where the 'film' shows much improved superconducting properties [13] , the enhanced superconducting properties of our epitaxial NbC films can come from the lattice strain, the inclusion of second phases, and/or the related defects during the growth. Figure 4: Superconducting properties of CNT–NbC composite. ( a ) Resistivity versus temperature characteristics at different applied magnetic fields, where the magnetic field is parallel to the CNT growth direction, ( b ) irreversibility field and upper critical field as a function of temperature obtained from those curves, where the irreversibility field H irr is defined as the field at which the ρ / ρ N =3% and the upper critical field as the field at which the ρ / ρ N =80%. Full size image A second important effect is that the superconducting properties of the CNT–NbC composite become anisotropic compared with pure NbC. 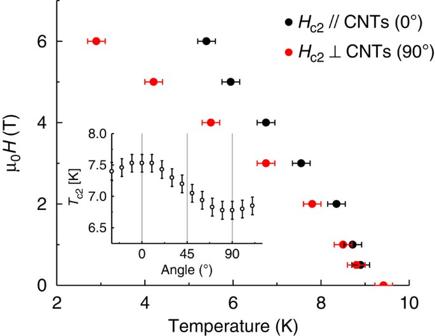Figure 5: Anisotropic properties of the upper critical magnetic field tested for another CNT–NbC composite. The inset shows the angular dependence of theTc2(the temperature at whichρ/ρN=80%) at an applied field of 3 T, where 0° and 90° correspond to the field parallel and normal to the CNT growth direction, respectively. Figure 5 shows the H c2 ( T ) for another CNT–NbC sample, where the H c2 ( T ) is obtained from resistivity versus temperature curves at different magnetic fields. It is apparent that H c2 ( T ) is higher when H is parallel to the aligned CNT forests than when it is perpendicular to them. The inset shows the angular dependence of the transition, T c2 (ΘΘ), at H =3 T. We can estimate the anisotropy as γ ~ H c2 (//CNT)/ H c2 ( CNT)~1.5. Figure 5: Anisotropic properties of the upper critical magnetic field tested for another CNT–NbC composite. The inset shows the angular dependence of the T c2 (the temperature at which ρ / ρ N =80%) at an applied field of 3 T, where 0° and 90° correspond to the field parallel and normal to the CNT growth direction, respectively. Full size image The enhanced H c2 implies a shorter superconducting coherence length ( ξ ). This is consistent with a reduction in the electronic mean free path ( l ) due to the increased disorder, which turns the material towards the 'superconducting dirty limit' and reduces the effective ξ (ref. 14 ). As the properties should be isotropic within the plane perpendicular to the CNT, for H //CNT, we can use ; so for T ~5 K, we obtain (ref. 12 ), where Φ 0 is the magnetic flux quantum. For H //CNT, we have ; thus, at T ~5 K, we estimate . The fact that may be a consequence of l in this direction not being constrained by the electron scattering with the CNT. Similarly to the strong correlated pinning in high-temperature superconducting YBCO crystals produced by aligned columnar defects created through high-energy heavy ion irradiation [7] , or in YBCO films by self-assembled second phase BaZrO 3 (refs 9 , 10 ), it is reasonable to speculate that the aligned CNT forests embedded in the superconducting NbC can function as effective correlated pinning centres for the vortices in the NbC. Moreover, in the CNT–NbC composite, we can not only maintain well-aligned CNTs, but also well-controlled diameter of the CNTs around 12±2 nm as shown in the Figure 2 . This diameter is well suited to pin vortices in NbC, as it is similar to the diameter of the vortex core, (ref. 15 ). In high-temperature superconductors such as YBCO, the irreversibility field H irr is associated with a thermodynamic solid–liquid phase transition in the vortex lattice. In the particular case of aligned columnar defects, a Bose–glass transition with a maximum in H irr for defects is observed [15] . In contrast, the lower T c and larger in the CNT–NbC composite result in a Ginzburg number Gi ~10 −7 , several orders of magnitude smaller than in YBCO; thus, an extended vortex liquid phase is not expected [12] and H irr just reflects pinning effects. This is consistent with the absence of broadening in the resistivity versus temperature characteristics with increasing H , as seen in Figure 4a . In contrast to the case of columnar defects introduced in anisotropic high-temperature superconductors, in the CNT–NbC composite both the anisotropy in H c2 and the vortex pinning are induced by the CNT; thus, detailed studies of the angular dependence of the critical current density below the H irr ( T , ΘΘ) line will be necessary to elucidate the pinning mechanisms. It should be noted that the area density of columnar defects is another important parameter one has to optimize to effectively pin the flux lines [7] . As the area density of the CNT forest is around 10 10 –10 11 cm −2 , corresponding to relatively low matching fields (B Φ , the field at which the density of vortices and defects are the same) of 0.2–2 T, we believe that we still have room to optimize the CNT volume density in the CNT–NbC composite. For example, we can manipulate the diameter of the CNTs as well as the area density of the CNT in the forest by controlling the layer thickness of the catalyst and the growth temperature of the CNT forests. We would like to point out that the results demonstrated here may not be directly applied to mixers and cavities. For example, an enhancement of conductivity through percolation normal to the CNT growth direction would not be expected to be achieved. However, an enhanced conductivity would be expected along the CNT growth direction because the CNTs are continuous from the top to the bottom of the forest. As a comparison, a resistivity of 70 μΩ cm was reported for NbC single crystals [16] . Our epitaxial NbC film has a resistivity of 60 μΩ.cm at 20 K (ref. 17 ). The resistivities for the CNT–NbC composite in this work are ~145 and ~110 μΩ cm normal and parallel to the CNT growth direction, respectively. More efforts are needed to apply CNT–NbC composites developed here for hot-electron bolometric superconducting mixers [3] and superconductive radio-frequency cavities [4] . However, the process developed here is adaptable for the synthesis of other format of CNT–NbC composites. We have recently demonstrated that polymer-assisted deposition can be used to grow high-performance superconducting NbC films [17] . It is possible that one can use the process developed here to coat NbC on CNT ribbons, if one can successfully pull CNT ribbons and attach them on a substrate. Therefore, the much improved superconducting properties achieved by forming CNT–NbC composites could be the first step towards potential new applications where mechanical strengths and high performance superconducting properties are required. In summary, we have demonstrated that well-aligned CNT forest can be embedded into superconducting NbC matrix, where CNTs can function as the effective vortex pinning centres. The CNT–NbC composite shows much enhanced and anisotropic H c2 and irreversibility field (5 T at 4.2 K). These values are far higher than those reported for the bulk NbC and other NbC combinations. Preparation of precursor Nb solution The precursor used for the deposition of NbC was an aqueous solution of Nb ion bound to polyethyleneimine. To prepare such a homogeneous solution, high purity (>99%) NbCl 5 , NH 4 OH, and 20% HF were dissolved in water, where the water was purified using the Milli-Q water treatment system. Ultrafiltration was carried out under 60 psi nitrogen pressure using Amicon-stirred cells that have a 3,000 molecular weight cutoff. In details, 2 g of NbCl 5 were converted to Nb(OH) 5 by adding ammonium hydroxide into the solution. The Nb(OH) 5 was then dissolved in 30 ml of deionized water and 7.5 ml of 20% HF. Polyethyleneimine was then added in 30 g aliquots (total 3.0 g) and mixed after each addition. After stirring, the solution was placed in an Amicon filtration unit designed to pass materials with molecular weight <30,000 g mol −1 . The solution was diluted 3 times to 200 ml and then concentrated to 35 ml in volume. Inductively coupled plasma-atomic emission spectroscopy showed that the final solution was 400 mM Nb. Synthesis of aligned carbon nanotube forests The CNT forests were synthesized by a chemical vapour deposition in a quartz tube furnace. The catalyst used for the growth of CNTs was a thin layer of Fe (~1.0 nm) deposited on Al 2 O 3 (~10 nm)/SiO 2 (~1 μm)/Si wafers. Forming gas (Ar+6% H 2 ) was used as carrier gas, and ethylene served as carbon source. The reaction was carried out at 750 °C for 120 min with 140 sccm forming gas and 30 sccm ethylene. The length of synthesized CNTs is around 0.6 mm. Coating NbC on highly aligned carbon nanotube forests The CNT–NbC composites were formed through thermal reaction under controlled environment. As-synthesized CNT forests were soaked by the Nb precursor solution. After the solution was permeated into CNT forests, the CNT forest was detached from the Si wafer simply by peeling off the CNT forest from the Si substrate using a tweezer. The CNT forests containing Nb precursor solution were heated to 650 °C at a rate of 10 °C min −1 in the mixture gases of ethylene (10 sccm) and forming gas (10 sccm). The sample was annealed at 650 °C under such an environment for 1 h. The mixture gases were switched to Ar (10 sccm) while the furnace was ramped to 1,000 °C in 1 h. The sample was annealed at this temperature in Ar for 3 h. Finally, the sample was naturally cooling to room temperature by turning off the power supply to the furnace. The thickness of synthesized CNT–NbC composite is close to 0.6 mm, which is similar to the length of CNT forest. Characterization The Nb concentration in the precursor solution was measured using a Horiba Jobin Yvon Ultima II inductively coupled plasma-atomic emission spectrometer. X-ray diffraction was used to characterize the crystallographic structure of the samples. The morphologies and microstructures of the samples were analysed by SEM and HRTEM. The resistivity versus temperature characteristics were measured using a standard four-probe technique by a Quantum Design Physical Properties Measurement System. How to cite this article: Zou, G.F. et al . Highly aligned carbon nanotube forests coated by superconducting NbC. Nat. Commun. 2:428 doi: 10.1038/ncomms1438 (2011).